The first archaicHomofrom Taiwan Recent studies of an increasing number of hominin fossils highlight regional and chronological diversities of archaic Homo in the Pleistocene of eastern Asia. However, such a realization is still based on limited geographical occurrences mainly from Indonesia, China and Russian Altai. Here we describe a newly discovered archaic Homo mandible from Taiwan (Penghu 1), which further increases the diversity of Pleistocene Asian hominins. Penghu 1 revealed an unexpectedly late survival (younger than 450 but most likely 190–10 thousand years ago) of robust, apparently primitive dentognathic morphology in the periphery of the continent, which is unknown among the penecontemporaneous fossil records from other regions of Asia except for the mid-Middle Pleistocene Homo from Hexian, Eastern China. Such patterns of geographic trait distribution cannot be simply explained by clinal geographic variation of Homo erectus between northern China and Java, and suggests survival of multiple evolutionary lineages among archaic hominins before the arrival of modern humans in the region. Palaeoanthropology in the 20th century established the long-time persistence of Homo erectus in the Pleistocene of Java and China, as well as the presence of a more encephalized form of archaic Homo in China and India. Recent studies emphasize some degree of regional and chronological variation within Asian H. erectus [1] , [2] , [3] , [4] , [5] , [6] , [7] , dismissing the previous claim that this species was an example of evolutionary stasis [8] , [9] . Furthermore, the diversity of archaic Asian hominins is highlighted by the discovery of a diminutive species, H. floresiensis , that evolved in isolation on the East Indonesian island of Flores from as early as ~1.0 million years ago [10] , [11] ; genetic evidence indicates that during the Late Pleistocene Neanderthals ranged from Europe to as far east as the Russian Altai in Southern Siberia [12] , [13] ; The discovery of ancient DNA distinct from both Neanderthals and modern humans has even led to the proposal of a new population, the ‘Denisovans,’ from Denisova Cave in the Altai [14] . Still, much of eastern Asia remains unsearched for fossil evidence of hominin occupation. Clearer documentations of morphological variations based on more fossil materials are essential to understand human evolution in this region. The new hominin mandible we describe here contributes to fill this geographic gap of the Asian fossil record. Penghu 1 (Access No. NMNS006655; Catalogue No. F051911; Repository, National Museum of Natural Science, Taichung) that was dredged by a fishing net from the −60 to −120 m deep Penghu submarine channel, 25 km off the western shore of Taiwan, together with other vertebrate fossils known as the terminal Middle/Late Pleistocene ‘Penghu fauna’ [15] , [16] ( Fig. 1 ; Supplementary Fig. 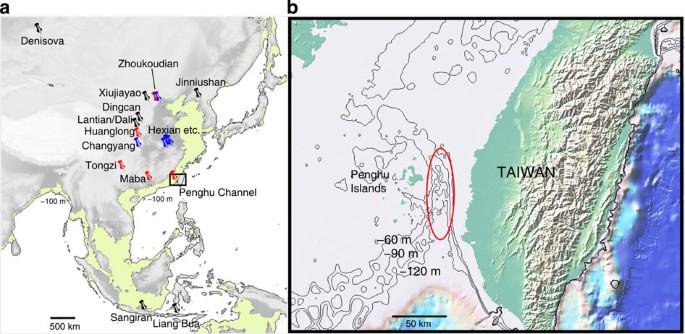Figure 1: Map of the major hominin sites mentioned in the text and the submarine topography around the Penghu Channel. (a) Map of the major hominin sites mentioned in the text. The red pins indicate the occurrence ofCrocuta crocuta ultima, and the blue pinsPachycrocuta brevirostris sinensis. The light green areas are the continental shelves 0–100 m below sea level. ‘Hexian etc.’=Hexian, Chaoxian and Tangshan. (b) The submarine topography around the Penghu Channel. The location of vertebrate fossil concentration in the Penghu Channel is encircled. The base map created using the GeoMapApp software (http://www.geomapapp.org/) and Global Multi-Resolution Topography synthesis69. 1 ; Supplementary Table 1 ; Supplementary Notes 1 and 2 ). The channel had been a part of the Asian mainland during episodes of Pleistocene low sea-level [17] . Because its stratigraphic context is unknown, the age of Penghu 1 can only be determined by analyzing the fossil specimen itself. In this paper, we report dating of Penghu 1 and discuss its evolutionary significance through morphological comparisons with other Pleistocene Homo from Africa, Europe and Asia. Figure 1: Map of the major hominin sites mentioned in the text and the submarine topography around the Penghu Channel. ( a ) Map of the major hominin sites mentioned in the text. The red pins indicate the occurrence of Crocuta crocuta ultima , and the blue pins Pachycrocuta brevirostris sinensis . The light green areas are the continental shelves 0–100 m below sea level. ‘Hexian etc.’=Hexian, Chaoxian and Tangshan. ( b ) The submarine topography around the Penghu Channel. The location of vertebrate fossil concentration in the Penghu Channel is encircled. The base map created using the GeoMapApp software ( http://www.geomapapp.org/ ) and Global Multi-Resolution Topography synthesis [69] . Full size image Dating Radiocarbon dating failed due to a lack of collagen and laser-ablation U-series dating had limited success because of uranium overprint in the seawater ( Supplementary Fig. 2 ; Supplementary Tables 3 and 4 ; Supplementary Note 3 ). To examine relative chronology of the Penghu fauna and Penghu 1 hominin mandible, we analyzed the contents of fluorine (F) and sodium (Na) in bone samples. F derives from surrounding soil and groundwater and accumulate slowly with time in apatite crystals of buried bones at the cost of hydroxyl ions [18] , [19] , [20] , [21] . Na, mostly surface bound in apatite crystals, exists about 1% in living bone [22] , [23] , [24] , [25] but tends to decrease in older, fossilized bones [22] , [23] , [24] . The contents of these elements relative to apatite in a fossil bone, which can be expressed as F/P 2 O 5 and Na 2 O/P 2 O 5 , respectively, are functions of factors reflecting its deposition history, such as the nature of the deposits, groundwater and the time passed since the burial. Therefore, similarities of these variables suggest similar depositional histories, and thus similar ages of the bones. We analyzed Penghu 1, as well as 20 Penghu fossil bones derived from 8 large-to-medium-bodied mammal taxa ( Palaeoloxodon , Bubalus , Sus , Elaphurus davidianus , Cervus , Equus ferus , Ursus arctos and Crocuta crocuta ultima : Supplementary Table 5 ). Because C. c. ultima is a useful biochronological guide taxon in eastern Asia [16] ( Supplementary Note 2 ), our primary interest is contemporaneity of Penghu 1 with this hyaenid. A bone sample of C. c. ultima was divided into two pieces to repeat the measurements. 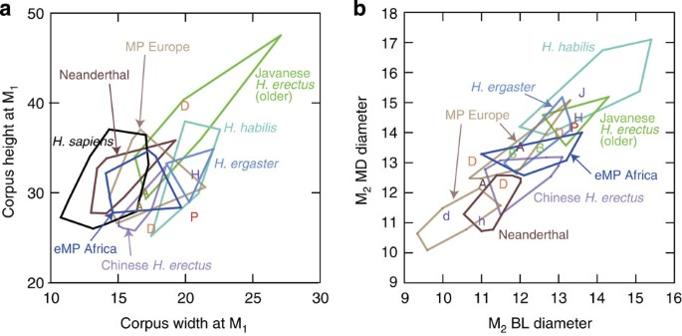Figure 5: Bivariate plots of selected measurements. Dimensions of mandibular corpora (a) and crowns of mandibular second molar (b) (in mm). Polygons indicate ranges when the sample size >3. The dental metrics of the MP European sample is divided into the smaller group (Atapuerca-SH) and the rest of it. Symbols: A, late EP EuropeanHomo(Atapuerca); B, Sangiran Upper (younger EP JavaneseH. erectus); D, Dmanisi; d, Dingcun; H, Hexian; h, Huanglong Cave; P, Penghu; S, Sangiran lower (older EP JavaneseH. erectus). The mean F/P 2 O 5 and Na 2 O/P 2 O 5 values are plotted in Fig. 2 . The variation seen in this figure probably reflects more or less diverse deposition histories and ages for individual bones from the Penghu Channel. The comparatively higher F/P 2 O 5 and lesser Na 2 O/P 2 O 5 values for the C. c. ultima samples suggest that this Crocuta individual is among the oldest of the Penghu faunal assemblage. The positions of Crocuta and Penghu 1 are close to each other, or Penghu 1 is slightly lesser in F/P 2 O 5 and higher in Na 2 O/P 2 O 5 contents than the Crocuta specimen. 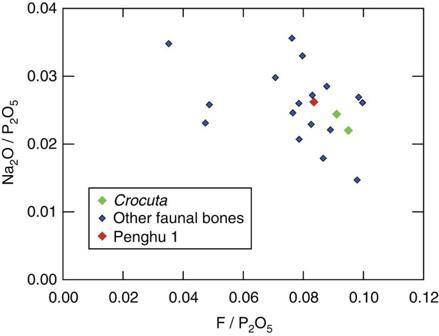Therefore, Penghu 1 is nearly contemporaneous with C. c. ultima or slightly postdate it. Figure 2: Plot of the relative F and Na contents in the bone samples from Penghu Channel. Slightly less F/P2O5and slightly greater Na2O/P2O5contents of Penghu 1 compared with those for theCrocutasamples suggest equal or slightly younger relative age for the former. Figure 2: Plot of the relative F and Na contents in the bone samples from Penghu Channel. Slightly less F/P 2 O 5 and slightly greater Na 2 O/P 2 O 5 contents of Penghu 1 compared with those for the Crocuta samples suggest equal or slightly younger relative age for the former. Full size image Morphology Penghu 1 is a nearly complete right side of the mandible with intact but extensively worn premolars and molars in place ( Fig. 3 ). The alveoli for the four incisors and right canine are preserved. The coronoid process is broken. Otherwise, the hemi-mandible is complete with no postmortem deformation or surface abrasion. No sign of pathology can be discerned. Although the M 3 was congenitally absent, the associated symptoms of malformation syndromes or systemic diseases (agenesis, microdontia, abnormal positions, enamel hypoplasia and so on) [26] , [27] are not evident. This specimen preserves a number of taxonomically diagnostic features despite being represented by a single skeletal element. Morphological descriptions of Penghu 1, comparative samples and their measurements are given in Supplementary Notes 4–6 and Supplementary Tables 6–9 . 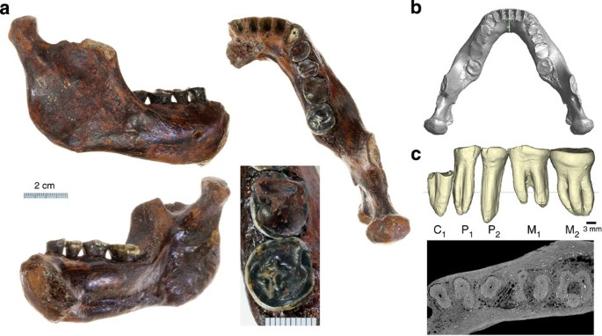Below, major characteristics of Penghu 1 are summarized to examine its taxonomic affinities. Figure 3: Penghu 1 mandible. (a) Mandible, (b) its virtual reconstruction and (c) surface rendered image of the segmented mandibular dentition (upper, lingual view) and its horizontal micro-CT section at the level indicated by the dotted line (lower). Figure 3: Penghu 1 mandible. ( a ) Mandible, ( b ) its virtual reconstruction and ( c ) surface rendered image of the segmented mandibular dentition (upper, lingual view) and its horizontal micro-CT section at the level indicated by the dotted line (lower). Full size image Penghu 1 is distinguished from H. sapiens by its strongly receding anterior surface of the mandible with no chin. It is derived relative to Australopithecus and early forms of Homo ( H. habilis and Dmanisi Homo ) in the short and relatively wide shape of its mandibular/dental arcade ( Fig. 4a–e ) [28] , [29] . 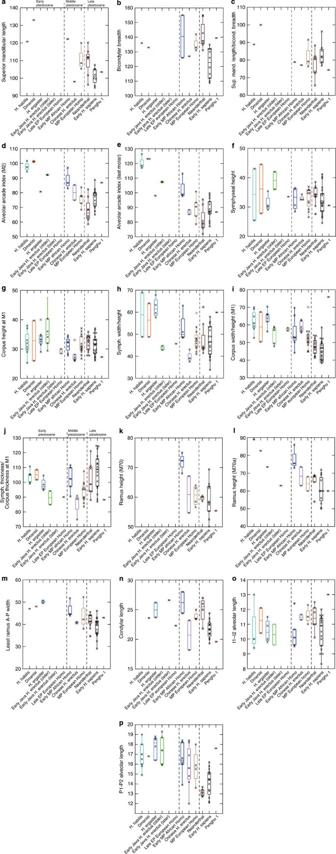This trait as well as an anteriorly extensive superior transverse torus [30] and M3 agenesis ( Supplementary Note 7 ) justifies the assignment of Homo to this specimen. Figure 4: Box plots of mandibular and dental arch metrics (mm) and ratio (%). Symbols give the median (horizontal line inside the box), central 50% range (box margins), range (vertical line) within inner fences (1.5 times box range from box margins) and outliers (asterisk). Each cross represents an individual specimen. The Penghu 1 mandible is short and moderately wide (a–c). Because M3failed to develop in Penghu 1, its alveolar arcade index measured at distal M2was compared with both the index at distal M2(d) and that at the last molar (e) for the comparative specimens. Although it is uncertain which comparison is more appropriate over the other, in either case, the arcade of Penghu 1 is wider thanH. habilis, Dmanisi and older JavaneseH. erectus. The mandibular body of Penghu 1 is low (f,g), but its robusticity indices are moderately or extremely high at the symphysis (h) and lateral corpus (i), respectively. Penghu 1 is more similar to the African and some European Early-Middle PleistoceneHomomandibles rather than to Javanese and ChineseH. erectusin these respects. On the other hand, Penghu 1 is closer to AsianH. erectusshowing relatively thinner symphyseal width as compared with lateral corpus width (j). Ramus height of Penghu 1 is, when two different measurements are considered together (k,l), considerably lower compared with the Early-Middle Pleistocene AfricanHomoand closer to EurasianHomospecimens from the late Early to Late Pleistocene contexts. The antero-posterior width of the ramus (m) of Penghu 1 is also lesser compared with the African and Georgian mandibles, but is slightly larger than or comparable to the medians for the Middle-Late Pleistocene Eurasian samples. The medio-lateral condylar length (n) is extremely small and comparable to one of the Zhoukoudian mandibles (Mandible H1) and to the smallest range forH. sapiens. The incisal portion of Penghu 1 is extremely wide (o). Only one of theH. habilis(rudolfensis) specimens (KNM-ER 60000 (ref.70) matches this Penghu 1 condition. The premolar portion is also extensive in Penghu 1 (p). Figure 4: Box plots of mandibular and dental arch metrics (mm) and ratio (%). Symbols give the median (horizontal line inside the box), central 50% range (box margins), range (vertical line) within inner fences (1.5 times box range from box margins) and outliers (asterisk). Each cross represents an individual specimen. The Penghu 1 mandible is short and moderately wide ( a – c ). Because M 3 failed to develop in Penghu 1, its alveolar arcade index measured at distal M 2 was compared with both the index at distal M 2 ( d ) and that at the last molar ( e ) for the comparative specimens. Although it is uncertain which comparison is more appropriate over the other, in either case, the arcade of Penghu 1 is wider than H. habilis , Dmanisi and older Javanese H. erectus . The mandibular body of Penghu 1 is low ( f , g ), but its robusticity indices are moderately or extremely high at the symphysis ( h ) and lateral corpus ( i ), respectively. Penghu 1 is more similar to the African and some European Early-Middle Pleistocene Homo mandibles rather than to Javanese and Chinese H. erectus in these respects. On the other hand, Penghu 1 is closer to Asian H. erectus showing relatively thinner symphyseal width as compared with lateral corpus width ( j ). Ramus height of Penghu 1 is, when two different measurements are considered together ( k , l ), considerably lower compared with the Early-Middle Pleistocene African Homo and closer to Eurasian Homo specimens from the late Early to Late Pleistocene contexts. The antero-posterior width of the ramus ( m ) of Penghu 1 is also lesser compared with the African and Georgian mandibles, but is slightly larger than or comparable to the medians for the Middle-Late Pleistocene Eurasian samples. The medio-lateral condylar length ( n ) is extremely small and comparable to one of the Zhoukoudian mandibles (Mandible H1) and to the smallest range for H. sapiens . The incisal portion of Penghu 1 is extremely wide ( o ). Only one of the H. habilis ( rudolfensis ) specimens (KNM-ER 60000 (ref. 70 ) matches this Penghu 1 condition. The premolar portion is also extensive in Penghu 1 ( p ). Full size image Both univariate ( Figs 4f–i and 5a ) and multivariate ( Fig. 6 ) analyses indicate that the low, thick body of the Penghu 1 mandible is more similar to some (but not all) of the ≥400 thousand years ago (ka) African (OH 13, 22; KNM-BK 8518), Georgian (D211) or European (Arago 13) Homo specimens rather than to our Early-Middle Pleistocene Asian sample (except Hexian discussed below). The corpus robusticity index (width–height ratio at M 1 : Fig. 4i ) of Penghu 1 (76%) is even greater than these robust non-Asian specimens (70%). Asian H. erectus mandibles from Zhoukoudian, Lantian and Sangiran all exhibit relatively thinner corpora (robusticity indices: 48–63%), and this also applies to Xujiayao 14, the sole existing archaic Homo mandible from 300–100 ka on mainland eastern Asia [31] ( Supplementary Note 5 ). However, Penghu 1 more closely resembles Asian H. erectus in a thinner symphysis relative to lateral corpus width ( Figs 4j and 6 ) and a lower and smaller mandibular ramus ( Fig. 4k–m ) that may be associated with the comparatively smaller and lower upper facial skeleton in archaic Asian Homo [32] . The condyle of Penghu 1 is very small, a character found only in a few specimens from the Zhoukoudian H. erectus or H. sapiens samples ( Fig. 4n ). Figure 5: Bivariate plots of selected measurements. Dimensions of mandibular corpora ( a ) and crowns of mandibular second molar ( b ) (in mm). Polygons indicate ranges when the sample size >3. The dental metrics of the MP European sample is divided into the smaller group (Atapuerca-SH) and the rest of it. Symbols: A, late EP European Homo (Atapuerca); B, Sangiran Upper (younger EP Javanese H. erectus ); D, Dmanisi; d, Dingcun; H, Hexian; h, Huanglong Cave; P, Penghu; S, Sangiran lower (older EP Javanese H. erectus ). 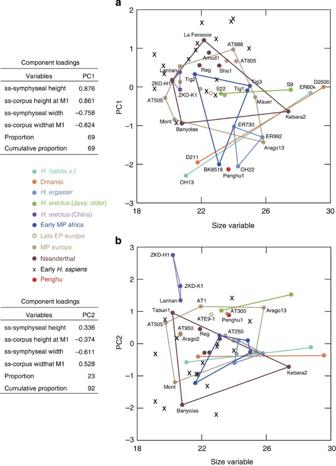Figure 6: Results of the PCA based on four size-standardized mandibular metrics. Scores for PC1 (a) and PC2 (b) against the ‘size variable’ (defined here as the geometric mean of the four measurements). Symphyseal height and width and corpus height and width at M1were used as the variables after divided by the size variable for each specimen. The principal component analysis (PCA) is based on the correlation matrix. Specimen names are indicated for archaic mandibles at least in one of the two figures. Those not indicated in either figure can be identified from the other figure because the two figures share thex-axis. The component loadings indicate that PC1, which explains 69% of the total variance, highly correlates with heights (positively) and thicknesses (negatively). PC2 explains 23% of the total variation, and tends to place those specimens with smaller symphyseal/lateral corpus thicknesses proportions on the positive side. The low PC1 score of Penghu 1 reflects its low and thick corpus. Irrespective of overall size of the corpus, Penghu 1 clusters with some of the Afro-EuropeanHomofrom the Early-Middle Pleistocene contexts (for example., OH 13, 22; KNM-BK 8518; D211; Arago XIII), but remote from AsianH. erectus, Neanderthals and earlyH. sapiens. In contrast, in PC2, Penghu 1 scores high together with AsianH. erectus, and is markedly different from African and Georgian Early-Middle Pleistocene mandibles. The score for Penghu 1 is around the highest end of variations exhibited by European archaic mandibles. Full size image Figure 6: Results of the PCA based on four size-standardized mandibular metrics. Scores for PC1 ( a ) and PC2 ( b ) against the ‘size variable’ (defined here as the geometric mean of the four measurements). Symphyseal height and width and corpus height and width at M 1 were used as the variables after divided by the size variable for each specimen. The principal component analysis (PCA) is based on the correlation matrix. Specimen names are indicated for archaic mandibles at least in one of the two figures. Those not indicated in either figure can be identified from the other figure because the two figures share the x -axis. The component loadings indicate that PC1, which explains 69% of the total variance, highly correlates with heights (positively) and thicknesses (negatively). PC2 explains 23% of the total variation, and tends to place those specimens with smaller symphyseal/lateral corpus thicknesses proportions on the positive side. The low PC1 score of Penghu 1 reflects its low and thick corpus. Irrespective of overall size of the corpus, Penghu 1 clusters with some of the Afro-European Homo from the Early-Middle Pleistocene contexts (for example., OH 13, 22; KNM-BK 8518; D211; Arago XIII), but remote from Asian H. erectus , Neanderthals and early H. sapiens . In contrast, in PC2, Penghu 1 scores high together with Asian H. erectus , and is markedly different from African and Georgian Early-Middle Pleistocene mandibles. The score for Penghu 1 is around the highest end of variations exhibited by European archaic mandibles. Full size image Penghu 1 lacks a suit of uniquely derived morphology of west Eurasian H. neanderthalensis (and in part its Middle Pleistocene predecessor, ‘ H. heidelbergensis ’), such as posteriorly located mental foramen and lateral prominence, an extensive retromolar space, a smoothly rounded gonial angle, a thin basal border of the ramus [33] and reduced postcanine teeth ( Figs 4p and 5b ). Metrically, Penghu 1 does not show antero-posteriorly elongated mandibular length that characterizes the Middle-Late Pleistocene European archaic mandibles (Mauer, Arago, most of the Neanderthals: Fig. 4a ). Compared with Penghu 1, these European specimens have higher and thinner bodies, higher rami and larger condyles, although one of them, Arago 13, approaches the Penghu condition in the body thickness as stated above. To examine tooth size, alveolar lengths were measured at the segments for incisors and premolars. The premolar length of Penghu 1 is large and comparable to those of the Early Pleistocene Homo ( Fig. 4p ), whereas the incisal length is the greatest among all the specimens compared here ( Fig. 4o ). A plot of the mesiodistal (MD) and buccolingual (BL) M 2 crown diameters ( Fig. 5b ) indicates that the Penghu M 2 (MD: 14.2 mm, BL: 13.4 mm) is comparatively large and is encompassed within the variations of the older Early Pleistocene Javanese H. erectus (the Sangiran Lower assemblage [29] ) and is similar to a specimen from Hexian ( Supplementary Note 8 ). It is at the largest ends of variations for Early-Middle Pleistocene post- habilis Afro-European Homo , and is distinctly larger than H. erectus from northern China and the terminal Early Pleistocene of Java (the Sangiran Upper assemblage [29] ). M 2 s are few from 300–50 ka of the mainland China, but at least reported such specimens from Dingcun and Huanglong Cave [34] , [35] are distinctly smaller than Penghu ( Fig. 5b ). Furthermore, none of the late archaic Chinese specimens (Jinniushan, Xujiayao, Chaoxian and so on dated to 280–30 ka; refs 34 , 36 , 37 , 38 , 39 ) exhibit large dimensions in M 2 ( Fig. 7b ) and I 1 ( Fig. 7a ) that probably mirror the trends in their mandibular antagonists (M 2 diameters ( Fig. 5b ) and I 1 –I 2 alveolar length ( Fig. 4o )). 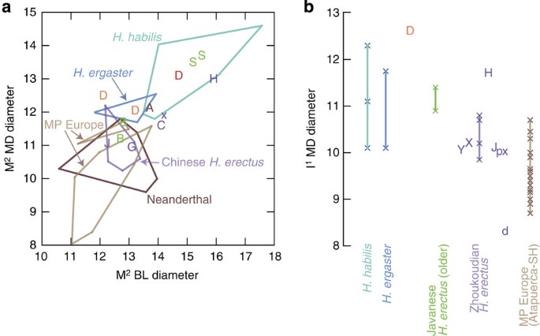Figure 7: Comparisons of the maxillary dental metrics (in mm). (a) Bivariate plot for M2. Polygons indicate ranges when the sample size >3. The dental metrics of the MP European sample is divided into the smaller group (Atapuerca-SH) and the rest of it. (b) MD diameters of I1. Sample ranges are shown by the coloured longitudinal lines with each cross indicating individual specimen. The two older Javanese EPH. erectusspecimens are Sangiran 7–85 and 7–86, whose reported stratigraphic levels are somewhat ambiguous31. Symbols: A, late EP EuropeanHomo(Atapuerca); B, Sangiran Upper (younger EP JavaneseH. erectus); C, Chaoxian; D (orange), Dmanisi; D (red), Denisova; d, Dingcun; G, Gongwangling (Lantian); H, Hexian; J, Jinniushan; p, Panxian Dadong; S, Sangiran Lower (older EP JavaneseH. erectus); X, Yunxian (Meipu); x, Xujiayao; Y, Yuanmou. Figure 7b also suggests that Penghu 1 is similar to ‘Denisovans’ [14] in M2 crown size; however, a direct comparison is not possible as there are no mandibles and mandibular teeth associated with this enigmatic Siberian hominin ( Supplementary Note 6 ). The root of the Penghu M 2 is unique: it is considerably longer than that of M 1 , and has a distinct extra root in between the lingual aspects of the mesial and distal roots ( Fig. 3c ). Figure 7: Comparisons of the maxillary dental metrics (in mm). ( a ) Bivariate plot for M 2 . Polygons indicate ranges when the sample size >3. The dental metrics of the MP European sample is divided into the smaller group (Atapuerca-SH) and the rest of it. ( b ) MD diameters of I 1 . Sample ranges are shown by the coloured longitudinal lines with each cross indicating individual specimen. The two older Javanese EP H. erectus specimens are Sangiran 7–85 and 7–86, whose reported stratigraphic levels are somewhat ambiguous [31] . Symbols: A, late EP European Homo (Atapuerca); B, Sangiran Upper (younger EP Javanese H. erectus ); C, Chaoxian; D (orange), Dmanisi; D (red), Denisova; d, Dingcun; G, Gongwangling (Lantian); H, Hexian; J, Jinniushan; p, Panxian Dadong; S, Sangiran Lower (older EP Javanese H. erectus ); X, Yunxian (Meipu); x, Xujiayao; Y, Yuanmou. Full size image Hexian, located 950 km north to the Penghu Channel on the Asian continent ( Fig. 1 ) is a hominin assemblage potentially similar to Penghu 1. Although the date of Hexian is controversial (~400–150 ka; refs 40 , 41 , 42 , 43 ) with the most recent combined ESR/U-series analysis supporting the older age [43] , the occurrence of Pachycrocuta brevirostris sinensis and the absence of C. c. ultima suggest that the site is older than Penghu ( Supplementary Note 2 ). The isolated incisor ( Fig. 7a ), premolar and molars from the assemblage are larger than northern Chinese H. erectus [44] , [45] , [46] , with a M 2 (PA839) similar to Penghu 1 in crown size and shape ( Fig. 5b ; Supplementary Note 8 ). The briefly described, fragmentary lateral mandibular corpus (PA831) from Hexian approaches the Penghu 1 condition in corpus width ( Fig. 5a ), although the former exhibits multiple mental foramina, a trait characteristic of Chinese H. erectus [29] , [34] . The above trace element analysis on the bone samples indicate that Penghu 1 is nearly contemporaneous with C. c. ultima from the same region or slightly postdate it. The fossil record at Zhoukoudian Locality 1 suggests that C. c. ultima appeared in northern China, between 250 and 500 ka (refs 47 , 48 ). However, a more primitive hyaenid taxon ( P. b. sinensis ) had persisted until later in Hubei (Changyang [49] , [50] (194–196 ka)), Anhui (Chaoxian [51] (160–200 ka), Hexian [41] (150–400 ka)), Jiangsu (Tangshan [52] (127–500 ka)) and other provinces in southern China ( Fig. 1 ; Supplementary Table 2 ; Supplementary Note 2 ). Sea-level lowering of >60 m occurred 10–70 and 130–190 ka during the past 240,000 years [53] . Penghu 1 probably deposited at the submarine channel during one of these phases by fluvial action. Older low-sea-level events, 225, 240–280, ?300, 335–360 and 425–450 ka [53] cannot be completely excluded as the age for Penghu 1, but such a situation requires explanation for preservation through repeated sedimentary events and the unusual distribution of C. c. ultima ( Fig. 1 ). Therefore, Penghu 1 is younger than 450 ka, and most likely 10–70 ka or 130–190 ka. Our morphological analyses show that Penghu 1 exhibits mosaic affinities with Chinese (small condyle), Asian (lower ramus, relatively thin symphysis), and non-Asian (low and thick corpus) archaic mandibles. It is also unique in its extremely large anterior tooth row and unusual M 2 root morphology ( Supplementary Table 9 ). Penghu 1 is most similar to Hexian, although their taxonomic affinities cannot be established without further comparative study and additional fossil discovery from the Penghu Channel. Hexian has been conventionally assigned to H. erectus but its large teeth and thick mandibular body demonstrated in this study and noted previously [44] , [45] , [46] , together with some unique cranial features [2] , urge further examination of its evolutionary relationships with the holotype or ‘classic’ H. erectus from Java and northern China [46] . Given this situation, at present it is difficult to assign species within the genus Homo for the new Taiwan mandible. Furthermore, the combination of the gracile (for example, corpus and ramus heights) and robust (corpus width and dental size) morphological elements in Penghu 1 makes sex determination difficult. The most striking observation derived from Penghu 1 is the unexpectedly late survival of the large teeth and thick mandibular corpus morphology in eastern Asia at least until ~400 ka but most likely beyond 190 ka ( Fig. 8 ). Several different models can be proposed to explain this situation. First, such morphology may be primitive retention from earlier Asian Homo . Because H. erectus mandibles from the terminal Early or early Middle Pleistocene of Java and China had already acquired thinner corpus and smaller molars [29] , this hypothesis implies the presence of another longstanding Homo lineage in Asia that continued from the Early Pleistocene. Otherwise, there may have been a migration of robust-jawed Homo from Africa, possibly bringing along Acheulean stone tool technology around the terminal Early Pleistocene [54] , who later evolved some unique morphology locally. Both hypotheses cast doubt on the traditional view that H. erectus was the sole hominin species on the Asian continent in the Early to early Middle Pleistocene, who exhibited clinal geographic variation across the continent from Indonesia to northern China [55] , [56] , [57] . The second model is compatible with but different from a recent suggestion that Chinese late archaic Homo received some genetic influence from west Eurasian Middle Pleistocene Homo [58] , and may be included in H. heidelbelgensis [59] , [60] . This is because Penghu 1 appears to be more primitive and similar to Hexian whose cranial morphology is distinct from Jinniushan and other late archaic Chinese Homo . Finally, the Penghu hominin may have evolved from a gracile-jawed local H. erectus population, but this is contrary to the general trend of dentognathic reduction in Pleistocene Homo [61] , [62] , [63] , which is documented even within the Early Pleistocene sequence of Sangiran, Java [29] , [64] , [65] . Whatever its origin was, this robust-jawed hominin highlights diversity of archaic occupants in the Middle-Late Pleistocene continental Asia before the appearance of H. sapiens 50–40 ka (refs 46 , 66 ). 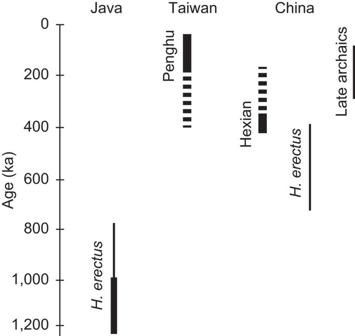Figure 8: Occurrence of thick mandibles and large M2s and I1s in Asia. Thick lines indicate the presence of these features. Chinese ‘late archaics’ are represented by Jinniushan, Xujiayao, Chaoxian and so on. Possible age ranges are indicated for Penghu and Hexian with their likely ages by solid lines. The occurrence of different hyaenid taxa (Pachycrocutaat Hexian andCrocutaat Penghu) suggest that Hexian predates Penghu. Figure 8: Occurrence of thick mandibles and large M2s and I1s in Asia. Thick lines indicate the presence of these features. Chinese ‘late archaics’ are represented by Jinniushan, Xujiayao, Chaoxian and so on. Possible age ranges are indicated for Penghu and Hexian with their likely ages by solid lines. The occurrence of different hyaenid taxa ( Pachycrocuta at Hexian and Crocuta at Penghu) suggest that Hexian predates Penghu. Full size image Trace element analysis To restrict the age of Penghu 1, we measured F and Na contents in the bones by an electron probe microanalyzer. The relative weight % of these elements were compared with those obtained from other mammalian fossils from the Penghu Channel, including C. c. ultima with known first appearance date in southern China. The cortical bone samples were cut by a thin diamond cutter. These trimmed samples were mounted using epoxy resin and polished before carbon coating. Then, the obtained flat surfaces were analyzed using an electron probe microanalyzer with the spot size of 3 μm. Natural fluoride (CaF 2 ), natural albite (NaAlSi 3 O 8 ) and synthetic mineral (P 5 DyO 14 ) were used as standards for F, Na and P, respectively. More than 30 spots at 0.1–0.2 mm intervals were randomly selected and measured, avoiding visible holes and cracks in the bone. A living bone contains about 38 wt% of P 2 O 5 (refs 18 , 67 , 68 ). We exclude those spots that have <30% P 2 O 5 contents in the following analyses as these results may be unreliable due to considerable foreign matter contamination. If F/P 2 O 5 or Na 2 O/P 2 O 5 values are outside the ranges of ±3 σ in each bone sample, such data are omitted as outliers. Supplementary Table 5 reports means and s.d. of F/P 2 O 5 and Na 2 O/P 2 O 5 for each bone sample after the above data selections. One of the specimens, F051720 ( Sus ), is distinct from the rest of the faunal samples showing unusually large variation in Na. Only three measurement values are available for F051695 ( Equus ). These two specimens are omitted in the comparison in Fig. 3 . Morphological analyses Penghu 1 was metrically and morphologically compared with most of the known Pleistocene Homo taxa, including H. habilis , H. ergaster , Middle Pleistocene African Homo , European Early and Middle Pleistocene Homo , Neanderthals, Indonesian H. erectus , Chinese H. erectus , post- erectus grade Chinese archaic Homo , early H. sapiens and others ( Supplementary Table 6 ). Comparative mandibular specimens were restricted to dentally adult individuals. The dental analyses focused on M 2 and anterior alveolar size, complemented by metrics for their maxillary antagonists. Due to the paucity of complete fossil mandibles and need to compare with the maximal available fossil samples including fragmentary specimens, metric analyses here are based on linear metrics. Dental root morphology was investigated by micro-computed tomogaryphy (CT) scan taken at the University Museum, the University of Tokyo, in 2010. Virtual reconstruction of Penghu 1 We reconstructed the entire mandibular shape of Penghu 1 ( Fig. 3b ) by mirror-imaging the polygon surface data of the complete right side derived from serial micro-CT images, using the Rapidform XOS software (INUS Technology, Seoul). We here defined the mid-sagittal plane as the plane passing through the infradentale and being perpendicular to both the alveolar plane and anterior tooth row: after defining the alveolar plane, the hemi-mandible was oriented in occlusal view perpendicular to it. Then a mirror image was made at the mid-sagittal plane defined above to reconstruct the left side of the mandible. It should be noted that this procedure does not perfectly reconstruct the basal symphysis of Penghu 1 because its symphyseal midline structures are slightly asymmetric; the above procedure is designed primarily to recover the original dental arcade shape and bycondylar breadth. To examine the error in determining the reference planes, the same procedure was repeated 1 month after the initial reconstruction. The two reconstructions were almost identical with 1.3 mm difference in the bicondylar breadth. The averages of the measurements taken from the two reconstructions were used for the present analyses. How to cite this article : Chang, C.-H. et al . The first archaic Homo from Taiwan. Nat. Commun. 6:6037 doi: 10.1038/ncomms7037 (2015).